Engineering colloidal quantum dot solids within and beyond the mobility-invariant regime Colloidal quantum dots are attractive materials for efficient, low-cost and facile implementation of solution-processed optoelectronic devices. Despite impressive mobilities (1–30 cm 2 V −1 s −1 ) reported for new classes of quantum dot solids, it is—surprisingly—the much lower-mobility (10 −3 –10 −2 cm 2 V −1 s −1 ) solids that have produced the best photovoltaic performance. Here we show that it is not mobility, but instead the average spacing among recombination centres that governs the diffusion length of charges in today’s quantum dot solids. In this regime, colloidal quantum dot films do not benefit from further improvements in charge carrier mobility. We develop a device model that accurately predicts the thickness dependence and diffusion length dependence of devices. Direct diffusion length measurements suggest the solid-state ligand exchange procedure as a potential origin of the detrimental recombination centres. We then present a novel avenue for in-solution passivation with tightly bound chlorothiols that retain passivation from solution to film, achieving an 8.5% power conversion efficiency. Colloidal quantum dots (CQDs) are nanocrystal semiconductor particles dispersed in solution that can readily be cast into electronically conducting solids. They enable bandgap tuning via adjustment of the nanoparticle size [1] , [2] . This has led to promising optoelectronic devices for lighting [3] , [4] , solar power conversion [5] , [6] , [7] , [8] , [9] and photon detection [10] , [11] . In solar cells, these materials have recently exceeded 7% certified power conversion efficiency (PCE) [5] , [12] , [13] , offering a promising path towards efficient, low-cost and roll-to-roll processed photovoltaics (PVs). Recent efforts have concentrated on eliminating trap states detrimental to carrier lifetime [5] , [14] , [15] , investigating the impact of size polydispersity on an ensemble of CQDs [16] , [17] , improving charge collection [13] , [18] , [19] , characterizing field-effect mobility in these materials [20] , [21] , [22] , [23] and developing novel doping strategies to enable new high-efficiency device architectures [6] , [24] , [25] , [26] . However, present-day devices still suffer from current densities and fill factors that are well below their theoretical potential. When employed as a PV material, a CQD solid must be strongly electronically coupled. This is facilitated in part by minimizing the nanocrystal spacing, enhancing charge carrier mobility [27] . In addition, it is desirable to eliminate surface-dangling bonds and chemical impurities to avoid formation of deep electronic trap states [5] , [28] that increase the rate of carrier recombination. If these features can be combined to produce a high mobility-lifetime product, increased transport lengths should permit the construction of thick absorber layers capable of absorbing the available solar light while maintaining the efficient harvesting of the resultant photocarriers. Despite numerous reports of field effect [23] , [29] , [30] and terahertz [22] , [31] mobilities on the order of 1–30 cm 2 V −1 s −1 , which should in principle result in much greater efficiencies than seen today [32] , a PV device has yet to be made that benefits from these increased charge carrier mobilities. Instead, the best certified CQD solar cells reported to date employ active layer materials with field-effect mobilities of 10 −3 –10 −2 cm 2 V −1 s −1 (refs 5 , 33 , 34 ). In this work, we demonstrate that present-day CQD PV materials are limited by the average recombination centre spacing within the film, which inhibits any gains to be made from an improved mobility. Diffusion length ( L D ) studies prompt the exploration of the disruptive ligand exchange procedure that is used for film fabrication as the culprit for the introduction of such recombination centres. Using a targeted strategy of in-solution passivation with chlorinated thiols to improve CQD protection during solid-state exchange, we achieve the reduction in trap densities, resulting in an 8.5% PCE using a standard planar device architecture. Charge transport regimes in CQD PV devices To shed light on the role of mobility in device operation, we first turn to a brief discussion of dominant transport modes in CQD PV devices. Charge carrier transport can occur in general by drift due to an electric field, or by diffusion. In the depleted heterojunction device employed in CQD PV ( Fig. 1a ), the energy bands of the p -type CQD solid (left) bend towards the interface with a highly n -type semiconductor electrode (right) such as TiO 2 . The doping level difference in the two materials is chosen to place the preponderance of the depletion region within the CQD solid. The resultant electric field enables efficient drift transport of photogenerated excess carriers at short-circuit conditions. 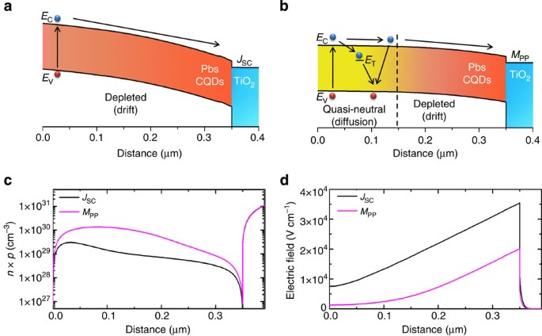Figure 1: Model and charge transport in CQD PV devices. (a,b) Energy-band diagrams of ap-type PbS CQD/n-type TiO2heterojunction shown at the (a) short-circuit condition and (b)MPPcondition. Electrons and holes are designated as blue and red spheres, respectively. (c,d) Simulated (c) electron-hole product and (d) electric field intensity as a function of position within the device. Figure 1: Model and charge transport in CQD PV devices. ( a , b ) Energy-band diagrams of a p -type PbS CQD/ n -type TiO 2 heterojunction shown at the ( a ) short-circuit condition and ( b ) M PP condition. Electrons and holes are designated as blue and red spheres, respectively. ( c , d ) Simulated ( c ) electron-hole product and ( d ) electric field intensity as a function of position within the device. Full size image To transfer not just current, but power, a load is placed across the p – n junction, lowering the built-in potential in the diode. At the maximum power point, M PP , depicted in Fig. 1b , the PbS CQD active layer is no longer fully depleted, and collection of photocarriers generated in the flattened band region now relies on diffusion. A minority carrier (electron) generated away from the depletion edge within the CQD layer may be collected, while carriers generated farther are more likely to be lost to recombination. Figure 1c shows the electron-hole ( n × p ) product for both the short-circuit condition ( J SC ) and M PP conditions, revealing charge carrier build-up in the quasi-neutral region for the M PP case, making these photocharges particularly prone to recombination. In addition, the electric field profiles in Fig. 1d show the shrinking of the depletion region and reduction of potential across the entire CQD layer. The photocurrent therefore diminishes as the device moves to M PP , which is reflected in a lowered fill factor. Achieving more efficient carrier extraction from the quasi-neutral region via enhanced diffusion will enable attainment of a notably higher fill factor, and will allow device thickness to be extended without compromise to other device parameters. Diffusion lengths in CQD PV materials Given the importance of the L D in CQD PV devices, we have developed a purely optical and contactless method to directly probe diffusion lengths rather than independently measuring mobilities and lifetimes. Typically, field-effect mobilities are obtained by raising the Fermi-level position by applying a gate voltage, filling in the intragap states and reducing the impact of traps. Diffusion length estimations based on combining these mobilities with lifetimes measured by other methods, thus, overestimate the diffusion length in the quasi-neutral region, misguiding the assessment of the material quality and hindering the identification of new paths towards improved CQD PV performance. We instead sought to measure the diffusion length directly. In the method employed, lifetime, mobility and effective trap density can also be extracted. We used donor/acceptor schemes employing different-bandgap CQDs in a layered one-dimensional approach, and separately in a mixed three-dimensional arrangement, and measured photoluminescence ratios between donor and acceptor emission to probe the radiative and transport-assisted non-radiative processes (details are provided in Supplementary Note 1 and Supplementary Fig. 1 ). The three-dimensional model accounts for the radiative and non-radiative decays within the CQD film ( Supplementary Fig. 2 ), and implements the acceptor phase as artificial traps to allow for the extraction of the trapping lifetimes and densities of recombination centres native to the donor phase, which are shown to inhibit the diffusion length ( Supplementary Note 2 ). The diffusion lengths were previously found to be ~30±10 nm for PbS CQDs capped with mercaptopropionic acid (MPA) in film and ~80±10 nm for the best previously reported CQD solids (hybrid CdCl 2 plus MPA passivation scheme [35] ). Multiple repeated trials allowed us to obtain the preceding uncertainty bounds, which arise from variations in film thickness and photoluminescence signal measurements. Our results and other recent publications on the subject yielding similar values [36] , [37] indicate that while the mobility was comparable in the two material classes, the trap density differed by a factor of three. This motivated us to undertake a closer inspection of these trap densities and their connection to diffusion lengths and transport in CQD solids. This would provide insight into the origins and methods of remedying these recombination centres. This work concentrates on the possibility that efficient transport of photocarriers to rare recombination centres could in fact dominate carrier loss [35] , [36] . Although L D depends on a mobility-lifetime product, the transport-assisted trapping lifetime can enter into a regime in which it is inversely proportional to mobility, rendering L D mobility invariant. In this regime, increasing the mobility further will simply allow the charge carrier to arrive at the trap faster, but will not affect its diffusion length. This is in contrast to a situation in which every dot has traps and the overall carrier lifetime is determined by the decay time within each dot [36] , [38] . In the latter case, improved mobility directly translates into improved diffusion length. In the presence of rare but detrimental traps, the diffusion length becomes limited by the average distance to the nearest deep trap. Specifically, we show ( Supplementary Note 3 ) that , where d is the dot-to-dot distance and N hops is the effective number of hops the carrier can make before encountering a trap. Equivalently, ( N hops ) −1 is proportional to the fraction of quantum dots that function as recombination centres. To illustrate these points, we plot ( Fig. 2a ) the effective lifetime as a function of mobility for several fixed trap densities, assuming a radiative lifetime of 1 μs. The effective lifetime decreases with increasing trap density and with increasing mobility. At low mobilities or trap densities, lifetime becomes limited by bandedge recombination. 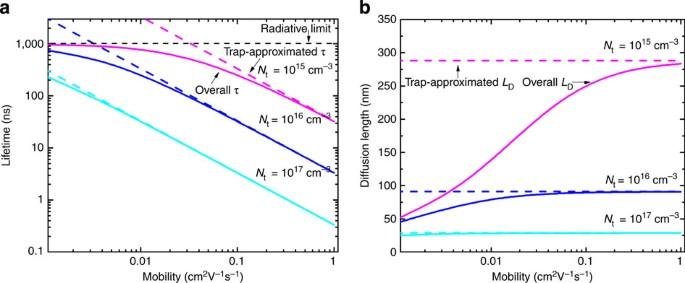Figure 2:Analysis ofLDparameters. Theoretical (a) lifetimes and (b) diffusion lengths for several mobilities and trap densities close to experimental values. Coloured dashed lines indicate parameter values obtained by considering only the trap lifetime. The radiative lifetime limit is also shown ina. Figure 2b shows the resulting L D plotted at different trap densities, where mobility is varied. For the trap densities around 10 17 cm −3 , L D is trap limited, and changing mobility does not affect the diffusion length. In this regime, traps are so common that carriers can reach and recombine within deep traps despite low mobility. As the trap density is decreased from today’s experimentally observed levels down to 10 15 cm −3 , diffusion lengths in the 150–250-nm range become possible. Further improving mobility above 10 −2 cm 2 V −1 s −1 can again have a pronounced effect on the improvement in L D , but it will again become trap limited for mobilities >1 cm 2 V −1 s −1 . Figure 2: Analysis of L D parameters. Theoretical ( a ) lifetimes and ( b ) diffusion lengths for several mobilities and trap densities close to experimental values. Coloured dashed lines indicate parameter values obtained by considering only the trap lifetime. The radiative lifetime limit is also shown in a . Full size image Device model with trap-limited L D To quantify the practical implications of our findings, we consider the impact of diffusion length on PV device performance in a conventional PbS/TiO 2 -depleted heterojunction [39] . In Fig. 3a we perform thickness-dependent measurements and observe the impact on FF, J SC and PCE. Since the depletion regions within these devices span only 100–200 nm (ref. 40 ), the thickness-dependent behaviour can reveal the role of the charge carrier diffusion length: J SC is expected to saturate once the thicknesses is increased beyond the sum of the depletion region thickness plus the diffusion length, and the fill factor will then also deteriorate owing to loss of depletion at the M PP . Experimentally, as the thickness is increased, J SC saturates and then slightly decreases due to increased series resistance, while the fill factor consistently decreases. Given this trade-off, the experimental PCE (shown in Fig. 3b ) is maximized at a thickness of ~300 nm, a quantity of CQD film not sufficient to absorb all incident above-bandgap solar radiation. 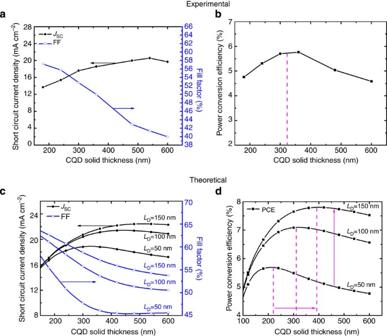Figure 3: Comparison of experimental and modelled PCE. Experimental (a)JSCand fill factor and (b) PCE for hybrid passivated CQD solids as a function of PbS active layer thickness. Theoretical simulations of (c)JSCand fill factor and (d) PCE for the PbS CQD/TiO2heterostructure device, for a range of different diffusion lengths. Magenta-dashed lines indicate PCE maxima, while red arrows indicate the increase in thickness (horizontal) and PCE (vertical) as longer diffusion lengths become accessible. Lines are drawn as a guide to the eye. Figure 3: Comparison of experimental and modelled PCE. Experimental ( a ) J SC and fill factor and ( b ) PCE for hybrid passivated CQD solids as a function of PbS active layer thickness. Theoretical simulations of ( c ) J SC and fill factor and ( d ) PCE for the PbS CQD/TiO 2 heterostructure device, for a range of different diffusion lengths. Magenta-dashed lines indicate PCE maxima, while red arrows indicate the increase in thickness (horizontal) and PCE (vertical) as longer diffusion lengths become accessible. Lines are drawn as a guide to the eye. Full size image We used the insights gained from our diffusion measurements to build a quantitative self-consistent optoelectronic model (see Methods) [41] , [42] . This, correlated with experimental work, permits analysis of avenues for further improvement in CQD PV performance. Figure 3c presents simulated depleted heterojunction devices where diffusion length was controlled by appropriately tuning the trap density, thus changing the lifetime. These studies quantitatively predict the trends seen in experiments. As expected, increased diffusion length allows for an increase in device thickness ( Fig. 3d ) according to the enhancement in L D . Improving the diffusion length by reducing the trap density will require more precise engineering of the CQD surface with the goal of a more complete passivation. Packing additional ligands onto the CQD surface or growing a complete shell to passivate the core more fully can be expected to improve overall charge carrier lifetimes [38] , [43] , [44] . In addition, unintentionally introduced impurities presented at the time of synthesis or deposition represent a little-explored potential source of midgap trap states [45] , [46] , [47] , [48] . Distinguishing the nature of trap states in these studies may be done spectroscopically [49] and with transmission electron microscopy [50] . The as-prepared films may be post treated with inorganic passivations—using methods such as atomic layer deposition [51] or successive ion layer adsorption and reaction [36] —to infiltrate the film and fully passivate any remaining bare surface sites. Another route to such a matrix could include fusing shell materials from core-shell nanoparticles via sintering [52] . Remarkably, the diffusion measurement technique used herein provides an estimate of a 10 16 cm −3 recombination centre density. This corresponds to roughly one deep detrimental trap per 1,000 nanocrystals; this is extremely rare considering the abundance of surface atoms in the CQD solid (~10 22 cm −3 ) and the fact that processing is carried out in an air ambient. This provides a hint that surface passivation might not be the only culprit in CQD film trap state densities, and prompted us to explore other possibilities for trap formation. For example, during solid-state fabrication, the often disruptive ligand exchange process may undo some of the excellent passivation afforded in solution, potentially causing nanocrystal fusion. Noticeably lower recombination centre densities in unexchanged CQD films [35] support this hypothesis. Hence, a single-step deposition approach, in which the final transport-compatible short ligand is administered during the solution-phase exchange, is attractive for reasons of prospective performance as well as of manufacturability [53] , [54] , [55] , [56] , [57] , [58] . Seeking to avoid the possibility of CQD fusion during the solid-state ligand exchange, we took an alternative approach, administering tightly bound thiols ( Fig. 4a ) in the solution phase with the idea that they could remain in place even during the disruptive ligand exchange process and, thus, avoid transiently unprotected CQDs. Experimental implementation using various short-chain thiols and particularly chlorinated propanethiols were rapidly screened by looking at solution photoluminescence quantum yield (PLQY), from which it was found that the thiolated CQDs have a higher PLQY ( Supplementary Fig. 3a ). Solution PLQY before versus after washing with methanol (a process known to remove excess surface ligands) remained stable for chlorothiol-treated CQDs, whereas it degraded noticeably for CQDs without thiols ( Supplementary Fig. 3b ), suggesting greater stability of chlorothiol-treated CQDs. This furthermore translated into improved PV performance, with benefits to all device parameters ( Supplementary Fig. 3c ), particularly fill factor (which is carrier diffusion related, as previously noted). X-ray photoelectron spectroscopy (XPS) revealed successful incorporation of the chlorothiol ligand that remained on the CQD surface after exchange ( Supplementary Fig. 4 ). 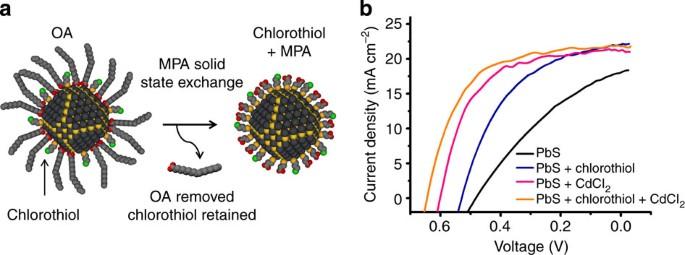Figure 4: Chlorothiol passivation scheme. (a) Premise of the chlorothiol passivation scheme employing tightly binding thiols that are retained during solid-state exchange. (b) RepresentativeJ–Vcurves of all materials classes comprising the layered passivation scheme employing the novel chlorothiol passivation approach. At least five devices were tested for each type of material. Figure 4: Chlorothiol passivation scheme. ( a ) Premise of the chlorothiol passivation scheme employing tightly binding thiols that are retained during solid-state exchange. ( b ) Representative J – V curves of all materials classes comprising the layered passivation scheme employing the novel chlorothiol passivation approach. At least five devices were tested for each type of material. Full size image J – V curves ( Fig. 4b ) under 1 sun illumination for the best obtained devices for each class of materials show that the sequential passivation strategy, with chlorothiols followed by a CdCl 2 treatment, yielded the best performance of 8.5%. Although previous optimization schemes achieved similar performance by exploiting improved electrode design [59] , this work does so through CQD solid engineering alone. Interestingly, chloro-propanethiol-treated CQDs can reach ~6% PCE on their own without any CdCl 2 treatment, compared with the ~3% obtained for the non-chlorothiol-treated CQDs. Ultimately, the combined passivation approach using chlorothiols in combination with CdCl 2 directly in solution enables superior PV performance, and will allow greater flexibility in obtaining trap-free colloidal nanocrystals and nanocrystal solids. This work suggests that, even at vastly subunity densities of recombination centres per quantum dot, the management of the CQD surface remains the most urgent frontier in CQD PV. On the basis of the optoelectronic device model developed in this work, we project in Fig. 5 that a moderate improvement of trap densities will lead to ~11% PCE, while reaching diffusion lengths of 1 μm will enable ~15% PCE. These projections assume continued improvements in both mobility and trap density over time, and also that film thicknesses can be substantially increased using the deposition methods available. Recent advances in perovskite solar cells, in which an order of magnitude improvement in diffusion length enabled drastic PCE improvements on a planar architecture [60] , are consistent with this view. Improvements in PCE beyond these projections will require addressing the suboptimal open circuit voltage values, currently observed in all types of solution-processed thin-film PV: CQDs [5] , perovskites [60] , copper indium gallium selenide (CIGS) [61] , copper zinc tin sulfide (CZTS) [62] and polymers [63] . 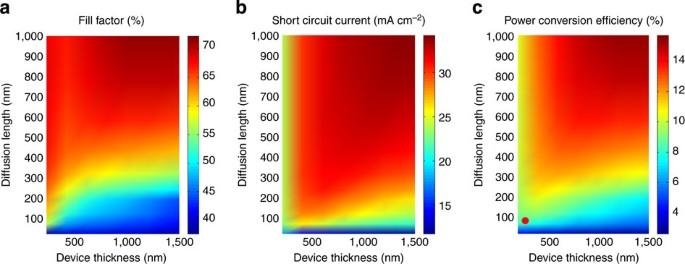Figure 5: Future performance projections based on optoelectronic model. Simulated (a) fill factor (b)JSCand (c) PCE for thickness up to 1.5 μm and diffusion lengths of 1 μm, showing that higher diffusion length will allow for increased device thickness and improved performance. The red dot represents best present-day performance. Figure 5: Future performance projections based on optoelectronic model. Simulated ( a ) fill factor ( b ) J SC and ( c ) PCE for thickness up to 1.5 μm and diffusion lengths of 1 μm, showing that higher diffusion length will allow for increased device thickness and improved performance. The red dot represents best present-day performance. Full size image Through this work, we have revealed the trap-limited, mobility-invariant regime and have identified and verified advanced routes to improved surface passivation, translating into record device performance on the most commonly employed electrode platform. Given the high extinction coefficients in CQD materials, active layer thicknesses and diffusion lengths on the order of 1 μm will allow closer approach to the Shockley–Queisser limit, and yield highly efficient and inexpensive solution-processed CQD PV. Materials preparation Organic-crosslinked and hybrid PbS CQDs of ~3 nm are fabricated following published recipes [2] . For chlorothiol-based CQDs, thiol treatment was performed during the cooling process. Chloropropane thiol concentration in the precursor was varied with octadecene. Thiol precursor (1.0 ml) was introduced into the reaction flask at 60 °C. Combination of thiol and cadmium precursor (CdCl 2 and tetradecylphosphonic acid at 13.8:1 molar ratio dissolved in oleylamine at 100 °C) treatment was made in two steps: thiol was injected first at ~100 °C and then Cd precursor was introduced into the reaction flask at 60 °C. The final PbS CQDs were isolated by addition of acetone (60 ml) followed by centrifugation after the reaction temperature reached 30–35 °C. The CQDs were then purified by dispersion in toluene and re-precipitation with acetone and re-dissolved in anhydrous toluene. The solution was washed with methanol three times with the final re-dispersion in octane at a concentration of 50 mg ml −1 . PV device fabrication PbS CQD films were deposited using a layer-by-layer spin-coating process under an ambient atmosphere. For each layer, the CQD solution (50 mg ml −1 in octane) was deposited on the ZnO/TiO 2 substrate and spin-cast at 2,500 r.p.m. Solid-state ligand exchange was performed by flooding the surface with 1% v/v MPA in methanol for 3 s before spin-coating dry at 2,500 r.p.m. Two washes with methanol were used to remove unbound ligands. Devices were made with variable-layer thicknesses. Top electrodes were deposited using an Angstrom Engineering Åmod deposition system in an Innovative Technology glovebox. The contacts typically consisted of 10 nm thermally evaporated molybdenum trioxide deposited at a rate of 0.2 Å s −1 , followed by electron-beam deposition of 50 nm of gold deposited at 0.4 Å s −1 , and finally 120 nm of thermally evaporated silver deposited at 1.0 Å s −1 . AM1.5 PV performance characterization Current–voltage data were measured using a Keithley 2400 source meter. The solar spectrum at AM1.5 was simulated to within class A specifications (less than 25% spectral mismatch) with a xenon lamp and filters (ScienceTech; measured intensity of 100 mW cm −2 ). The source intensity was measured with a Melles–Griot broadband power meter through a circular 0.049 cm 2 aperture at the position of the sample and confirmed with a calibrated reference solar cell (Newport). The accuracy of the current–voltage measurements was estimated to be ±7%. Device simulation SCAPS simulation software [41] , [42] was used. The software is available on contacting the software author directly. A full material parameter list is given in Supplementary Table 1 , with alpha coefficients in Supplementary Fig. 5 . The device structure was simulated from Fig. 1 of the main text. A solar spectrum excitation was used. Contact boundary conditions were specified as ohmic. Traps were introduced 0.2 eV below the conduction band as a single effective level, with capture cross-sections on the order of a 3-nm CQDs cross-sectional area, at a variable total density in the neighbourhood of 10 16 –10 17 cm −3 , corresponding to the diffusion lengths shown in Fig. 3 , which are readily calculated and reported within the simulation programme. For Fig. 5 , trap densities were reduced to 10 15 cm −3 , which corresponded to a lifetime of 1 μs within the simulator. Beyond this point, the mobility was used to tune the diffusion length to 1 μm. PLQY measurements PLQY measurements were performed in an integrating sphere using 1 mm cuvettes with a solution of optical density <0.1. The excitation source was a red 640 nm diode laser, and the detector used was a calibrated Ocean Optics USB2000 for the visible range along with an NIR512 for the near infrared. XPS measurements XPS was measured with a Thermo Scientific K-Alpha spectrometer to verify the incorporation of chlorothiols as ligands and their survival after solid-state ligand exchange. The core level spectra of Pb-4 f , S-2 p , O-1 s , C-1 s and Cl-2 p were measured with a pass energy of 150 eV. How to cite this article: Zhitomirsky, D. et al. Engineering colloidal quantum dot solids within and beyond the mobility-invariant regime. Nat. Commun. 5:3803 doi: 10.1038/ncomms4803 (2014).